Witnessing the formation and relaxation of dressed quasi-particles in a strongly correlated electron system The non-equilibrium approach to correlated electron systems is often based on the paradigm that different degrees of freedom interact on different timescales. In this context, photo-excitation is treated as an impulsive injection of electronic energy that is transferred to other degrees of freedom only at later times. Here, by studying the ultrafast dynamics of quasi-particles in an archetypal strongly correlated charge-transfer insulator (La 2 CuO 4+ δ ), we show that the interaction between electrons and bosons manifests itself directly in the photo-excitation processes of a correlated material. With the aid of a general theoretical framework (Hubbard–Holstein Hamiltonian), we reveal that sub-gap excitation pilots the formation of itinerant quasi-particles, which are suddenly dressed by an ultrafast reaction of the bosonic field. The exotic electronic ground states of transition-metal oxides (TMOs), such as high-temperature superconductivity and colossal magnetoresistance, arise from both the strong interactions among electrons and the complex interplay between the electronic and bosonic degrees of freedom such as lattice vibrations and magnetic excitations [1] , [2] , [3] , [4] . A prime example of such complexity is represented by the cuprate family. Starting from parent compounds which are charge-transfer (CT) insulators [5] , [6] , [7] , [8] , [9] , [10] , [11] , [12] , [13] , anomalous metallic and eventually high-temperature superconducting phases appear on electron or hole doping [14] , [15] . The properties of CT insulators are determined by Coulomb repulsion, which forces the electrons to localize, freezing charge fluctuations. In such a state, the coupling between localized fermions and bosonic excitations, which is mediated by charge dynamics, is naively expected to be strongly suppressed [16] , [17] . Although this scenario is seemingly met when we measure and study the properties of a steady-state Mott insulator, a different situation arises if the system is doped [18] , [19] , [20] or driven out of equilibrium [13] , [21] , [22] . In particular, the naive picture would suggest that if we try to excite the system by means of a pulse with photon energy smaller than the CT gap, because of strong electron correlations, we would observe little effect on the material as the localized carriers have no chance to change their state and, therefore, they have no means to couple to bosonic excitations. In our study, a completely different scenario emerges, in which a coupled boson-charge mode is excited leading to an effective renormalization of the CT gap. Note that in the following we use the general term ‘boson’. This is due to the fact that although the Hubbard–Holstein Hamiltonian (HHH) was developed to treat lattice vibrations, the same model can be used to address other kinds of bosonic excitations such as collective electronic modes. The punctual identification of these bosonic modes remains controversial in the cuprates and is beyond the scope of this paper. Further information can be found in refs 23 , 24 , 25 . Here, we show that a model including both local Coulomb interaction and coupling with a boson mode (HHH) accounts for our main experimental observations. The effects of the electron–boson coupling are highlighted by comparing the dynamical optical responses of La 2 CuO 4+ δ driven by pulses with photon energy respectively larger and smaller than the gap, which corresponds to the energy needed to create free charge excitations. Time-resolved measurements on La 2 CuO 4+ δ Transient reflectivity experiments on La 2 CuO 4+ δ were performed with above-gap (~3.1 eV) and sub-gap (~0.95 eV) ~100 fs long pump pulses and broadband probes as detailed in the Methods section. From the measured Δ R ( ω , τ )/ R ( ω )= R ( ω , τ )/ R ( ω )−1 with R ( ω , τ ), the time-dependent pump-perturbed reflectivity, and R ( ω ), the equilibrium reflectivity, we calculate the pump-induced changes of the optical conductivity Δ σ 1 ( ω , τ )= σ 1 ( ω , τ )- σ 1 ( ω ) as a function of probe frequency ( ω ) and pump–probe delay time ( τ ). Here, σ 1 ( ω , τ ) and σ 1 ( ω ) are the time-dependent light-perturbed and equilibrium optical conductivity, respectively. The CT peak (CTP) in σ 1 ( ω ) is at ~2.3 eV, while the gap, estimated from a simple linear interpolation (red dashed line in Fig. 1 ), is at about Δ=1.8 eV for T =130 K and is consistent with previous reports [6] , [7] , [8] , [9] , [26] . The non-vanishing optical conductivity below the gap is due to the presence of tail states. Such tail states originate from the strong interaction between the free charges in excess, coming from oxygen non-stoichiometry [23] , and the bosonic degree of freedom [13] . The excess oxygen content δ ~5 × 10 −3 is estimated from the measured Néel temperature of 229 K (ref. 27 ). Δ σ 1 ( ω , τ ) is obtained from Δ R ( ω , τ )/ R ( ω ) with a novel data analysis methodology based on the Kramers-Kronig (KK) relations. In short, by knowing the equilibrium reflectivity R ( ω ) and the non-equilibrium Δ R ( ω , τ )/ R ( ω ), it is possible to calculate the pump-perturbed reflectivity R ( ω , τ ) and, from it, all the transient optical properties (see Methods). 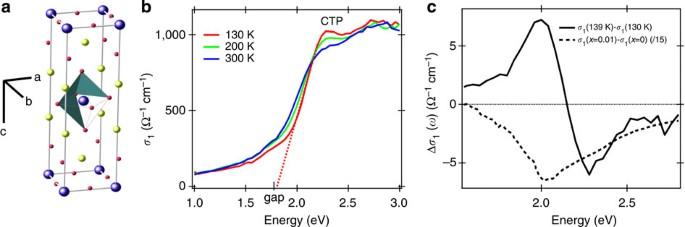Figure 1: Equilibrium optical conductivity of lanthanum-copper oxide for polarization in the oxygen plane. (a) La2CuO4unit cell with copper in purple, oxygen in red and, lanthanum in yellow. (b) In plane optical conductivity at 130 K, 200 K, and room temperature as determined via ellipsometry. The charge-transfer peak (CTP) is indicated. The red dashed straight line allows to define the gap at ~1.8 eV. (c) Expected variation ofσ1(ω) on doping (dashed line) or heating (solid line). The solid line is obtained from our ellipsometry data, the dashed line is the difference between the optical conductivity of La1.99Sr0.01CuO4(x=0.01) and La2CuO4(x=0) at room temperature. This last curve has been calculated starting from the data reported in ref.6. Specifically, to obtain thex=0.01 doping reported inc, we performed a linear interpolation between thex=0 and thex=0.02 spectra shown in ref.6. Figure 1: Equilibrium optical conductivity of lanthanum-copper oxide for polarization in the oxygen plane. ( a ) La 2 CuO 4 unit cell with copper in purple, oxygen in red and, lanthanum in yellow. ( b ) In plane optical conductivity at 130 K, 200 K, and room temperature as determined via ellipsometry. The charge-transfer peak (CTP) is indicated. The red dashed straight line allows to define the gap at ~1.8 eV. ( c ) Expected variation of σ 1 ( ω ) on doping (dashed line) or heating (solid line). The solid line is obtained from our ellipsometry data, the dashed line is the difference between the optical conductivity of La 1.99 Sr 0.01 CuO 4 ( x =0.01) and La 2 CuO 4 ( x =0) at room temperature. This last curve has been calculated starting from the data reported in ref. 6 . Specifically, to obtain the x =0.01 doping reported in c , we performed a linear interpolation between the x =0 and the x =0.02 spectra shown in ref. 6 . Full size image Temporal response The results reported in Fig. 2a,b are for pump pulses with photon energy at E pump =3.1 eV and E pump =0.95 eV, respectively, with ~0.04 eV pulse bandwidth each (see Methods for details). In the first hundred femtoseconds, we observe striking differences between the photo-excitation with photons at energy E pump >Δ ( Fig. 2a ) and E pump <Δ ( Fig. 2b ). A smooth rise time (>100 fs) is detected only for E pump >Δ, while sub-gap excitation leads to a pulse-width-limited rise time of the signal followed by an ultrafast decay. This difference is made evident in Fig. 2c , where the optical response at the CTP is shown as a function of the pump–probe delay. The results in Fig. 2c are normalized to the energy absorbed by the sample for E pump =3.1 eV (solid blue curve) and E pump =0.95 eV (solid red curve), respectively (see Methods for details). Although in a different physical context, it is worth mentioning here that ultrafast responses to an optical pump below the gap in multiple quantum wells [28] and below the electronic excitation energy in molecular systems [29] has been previously reported. 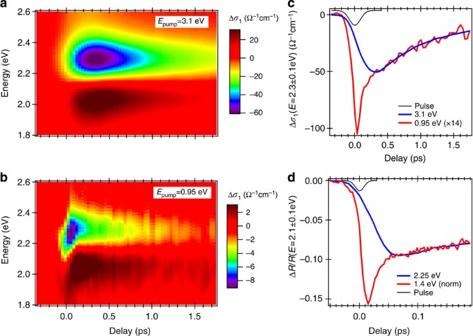Figure 2: Time-domain evolution of optical conductivity. The measurements performed at 130 K are reported as a function of probe energy for pump energy (a) larger (3.1 eV with 0.04 eV bandwidth) and (b) smaller (0.95 eV with 0.04 eV bandwidth) than Δ. (c) The transient optical conductivity atEprobe=2.3 eV for both pump energies is shown (3.1 eV in blue, 0.95 eV in red). The response for sub-gap excitation is multiplied by the ratio of the absorbed energy densities (see Methods). The black curve depicts the 3.1 eV pump autocorrelation. (d) Normalized pump–probe reflectivity measurements performed at room temperature with ~10 fs pulses (in black the pulse duration, see Methods for details). Figure 2: Time-domain evolution of optical conductivity. The measurements performed at 130 K are reported as a function of probe energy for pump energy ( a ) larger (3.1 eV with 0.04 eV bandwidth) and ( b ) smaller (0.95 eV with 0.04 eV bandwidth) than Δ. ( c ) The transient optical conductivity at E probe =2.3 eV for both pump energies is shown (3.1 eV in blue, 0.95 eV in red). The response for sub-gap excitation is multiplied by the ratio of the absorbed energy densities (see Methods). The black curve depicts the 3.1 eV pump autocorrelation. ( d ) Normalized pump–probe reflectivity measurements performed at room temperature with ~10 fs pulses (in black the pulse duration, see Methods for details). Full size image In Fig. 2c , we show that the modifications of the optical response at the CTP induced by the two stimuli are different in the initial dynamics while they become similar for longer delays between the pump and the probe pulses. As the data are normalized to the absorbed energy, the good agreement for large delays indicates that this ‘slow’ response is directly related to absorption, that is, to real electronic excitations. Such ‘slow’ response is consistent with previous time-resolved measurements on La 2 CuO 4 (refs 30 , 31 ), Nd 2 CuO 4 (refs 30 , 31 , 32 ), YBa 2 Cu 3 O y (ref. 32 ) and Sr 2 CuO 2 Cl 2 (ref. 21 ). Sub-20 fs pulse experiments With the aim to resolve the ultrafast rise time observed for E pump <Δ, we performed room temperature ~10 fs experiments with E pump <Δ (1.4 eV with 0.1 eV bandwidth) and E pump >Δ (2.25 eV with 0.25 eV bandwidth). In spite of the different excitation parameters used for the ~10 and ~100 fs measurements, we expect the outcome of these experiments to be meaningful for addressing the question concerning the non-thermal ultrafast rise time. The Δ R ( ω , τ )/ R ( ω ) at E probe ~2.1 eV is shown in Fig. 2d , while the transient reflectivity spectra at two pump–probe delays are reported in Supplementary Fig. 1 and Fig. 2d . It is evident that also for ~10 fs E pump <Δ pulses the ultrafast shift of the optical response is limited by the temporal resolution of the experiments ( Supplementary Fig. 1 ). Such result sets the upper limit of the timescale of the non-thermal response in La 2 CuO 4+ δ to 20 fs. Unfortunately, under the present experimental conditions, a direct quantitative comparison of the thermalization times between the ~100 and the ~10 fs excitations is not meaningful. In particular, the thermalization time is significantly shorter for ~10 fs excitations (see Fig. 2c,d ). We attribute this effect to the remarkably different conditions in terms of excitation density and spectral content of the pulses used in the experiments (see Methods). In the following, we will discuss only the spectral responses of the pump–probe data obtained with ~100 fs pump pulses where the linear response regime has been proven (see Methods). Energy-dependent response We now take advantage of the broadband probe and describe the spectral dependence of the transient response. The energy-dependent Δ σ 1 ( ω , τ ) at a delay time τ =0.05 ps averaged over ±0.05 ps ( τ =0.3 ps, averaged over ±0.1 ps) is reported in Fig. 3a,b for the two pump energies (blue for 3.1 eV and red for 0.95 eV pulses, respectively). 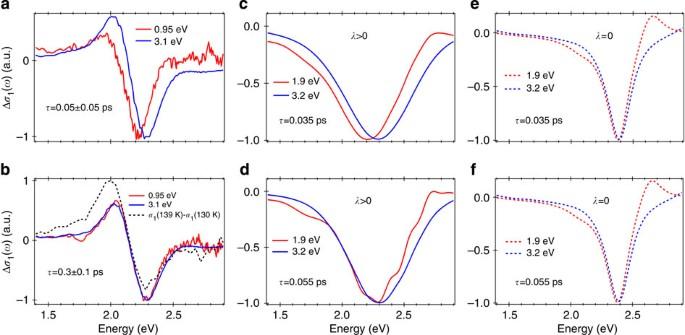Figure 3: Experimental and theoretical energy dependence of Δσ1at significant pump–probe delays. Inaandb, the experimental data are shown (the pulse bandwidth of about 0.04 eV is omitted in the labels); inc–f, the model calculations are reported. Ineandf, the zero-coupling results are reported for comparison. All the graphs share the same energy axis. The data are normalized for the sake of comparison. Figure 3: Experimental and theoretical energy dependence of Δ σ 1 at significant pump–probe delays. In a and b , the experimental data are shown (the pulse bandwidth of about 0.04 eV is omitted in the labels); in c – f , the model calculations are reported. In e and f , the zero-coupling results are reported for comparison. All the graphs share the same energy axis. The data are normalized for the sake of comparison. Full size image For E pump >Δ at both pump–probe delays, we observe a depletion of the optical absorption centred at E probe ~2.3 eV and an enhanced absorption around E probe ~2.1 eV. This behaviour can be ascribed to a ‘thermal response’, that is, it is compatible with the shift towards lower energies of the CTP on heating [27] , [30] , [31] as seen in Fig. 1 . This is confirmed by comparing the measured Δ σ 1 ( ω , τ ) at long pump–probe delays with the expected variation of the equilibrium optical conductivity for a temperature increase resulting from the pump-induced heating of the sample (black line in Fig. 3b , see Methods for details). On the contrary, Δ σ 1 ( ω , τ ) for E pump <Δ reveals a significant spectral evolution with time. The main feature remains an optical conductivity depletion around the CTP, but the energy dependence of the response depends on the pump–probe delay time τ . The Δ σ 1 ( ω , τ ) has a minimum at E probe ~2.2 eV within ~100 fs and drifts towards the thermal response only on longer times. It is important to notice that for τ ≤100 fs and E pump =0.95 eV the optical conductivity displays mainly a negative variation around E probe ~2.2 eV, which consists of an overall non-thermal quench of the CTP. This ultrafast variation of the optical conductivity resembles the one induced by small doping at equilibrium (see the dashed line in Fig. 1b ), that is, in both cases a broadband negative response at the CTP is present. To understand these experimental results, we now introduce the HHH. In the one-band Hubbard model, the optical gap for free charge excitations is related to the energy cost for unbound double occupancies (doublons). To explain the differences between the responses to sub-gap and above-gap excitations, one has to consider the two limiting cases predicted by time-dependent perturbation theory: non-adiabatic and adiabatic regimes. The non-adiabatic regime describes real transitions between electronic quantum states where the response is present for some time after the pump pulse is over. On the contrary, in the adiabatic regime the response comes from the deformation of the wave functions by the electric field of the light and the system comes back to the ground state when the pump pulse is over. Taking into account that the system is still out of equilibrium for several picoseconds after the pump pulse is over, we argue that the non-adiabatic contribution with real electronic transitions dominates the experimental response for E pump >Δ ( Fig. 2a ). Conversely, both contributions are essential for describing the dynamics for E pump <Δ. To describe the differences between the responses driven in La 2 CuO 4+ δ by sub-gap ( E pump =0.95 eV) and above-gap ( E pump =3.1 eV) ~100 fs long pump pulses ( Fig. 2 ), we turn to the HHH and introduce the effects of the electromagnetic fields through the classical vector potential A ( τ ) (see Methods). The HHH represents a standard approach for underdoped cuprates where the insulating state arises from the strong repulsion between the electrons. By taking into account both onsite Coulomb repulsion U and an effective electron–boson interaction [30] , the HHH can reproduce the equilibrium optical properties of cuprates both undoped and with tiny doping [13] and rationalizes the presence of tail states responsible for the broad below-gap absorption [13] , [27] , [33] . We argue that these tail states are responsible for the non-adiabatic contribution for sub-gap pumping and for the linearity of the optical response as a function of pump fluence (see Methods). Furthermore, we will show that the ultrafast transient optical response observed for E pump <Δ unveils a mixed regime of light–matter interaction where the light-driven gain of the electron kinetic energy leads to a sudden reaction of the bosonic field. As doping also drives a kinetic energy gain of the carriers, one naively expects an off-equilibrium ultrafast response similar to the one associated to doping at equilibrium (see Figs 1b and 3 ). The HHH is given by the sum of three terms: which account for the kinetic energy of the electrons (equation (1)), the onsite Coulomb repulsion (equation (2)) and the electron–boson interaction (equation (3)), respectively. In equations (1, 2, 3), t is the hopping amplitude, is the fermionic creation operator, μ is a lattice vector, creates a boson at site i with frequency ω 0 and n i is the electron number operator. The units are such that ħ =1. We choose model parameters typical for the cuprates ( t =0.3 eV, ω 0 =0.2 t , and the electron–boson coupling constant ). The value of the Hubbard repulsion U =10 t yields low-energy physics very similar to that of the t−J model with J =4 t 2 / U (see Methods). Although the exact solution for this Hamiltonian is not available, the time evolution of the many-body wavefunction | Ψ ( τ )› can be obtained in a small two-dimensional lattice (eight sites with periodic boundary conditions) by using an exact diagonalization method (time-dependent Lanczos approach) based on a smart truncation of the boson Hilbert space, which has been proven successful in different systems [34] , [35] . Spin and charge degrees of freedom are treated exactly within numerical precision. The optical conductivity is then calculated for a given value of the pump–probe delay τ , within the linear response theory, starting from the wave-function | Ψ ( τ )› (see Methods for more details). In Fig. 3c,d we show the calculated Δ σ 1 ( ω , τ ) at two different delay times both for above-gap (~3.2 eV) and sub-gap (~1.9 eV) ~40 fs long pump pulses. Please note that the slightly different pulse parameters used in the model compared with the experiment are required by the small lattice adopted in the calculations (see Methods). The major photo-induced feature calculated for E pump >Δ ( Fig. 3c,d ) is a reduction of the optical conductivity, which is consistent with the experiments ( Fig. 2a and Fig. 3a,b ). However, we observe quantitative discrepancies between the calculated linewidths and the measured ones. In particular, the calculated reduction of the optical conductivity extends over a broader energy range. We argue that this is due to the fact that the model is well suited to address doping phenomena [13] but lacks both the detailed crystal structure and a proper thermal reservoir. This interpretation is supported by comparing the expected variation of the optical conductivity on doping [6] (black dashed curve in Fig. 1b ) with the model results ( Fig. 3b ). Hence, for long pump–probe delays or E pump >Δ, the single boson mode contained in the HHH acts as an effective but quantitatively inaccurate thermal bath. Nonetheless, we stress that the theory accounts for the main experimental features and that a comparison between theory and experiment is fair, as both lie in the linear response regime (see Methods). In particular, both theory and experiments for E pump <Δ display a spectral response exhibiting an evolution on ultrafast timescales ( Fig. 3a–d ). We argue that such ultrafast changes of the spectral response are described by the model exclusively in the presence of strong electron–boson interaction, as can be seen by inspection of Fig. 3e,f that are obtained for electron–boson coupling λ =0. The ultrafast shift of the optical response for E pump <Δ may be rationalized as the result of a distortion of the bosonic field around holons and doublons [36] , [37] , leading to an energy renormalization close to the experimentally observed value [13] . In the following we discuss the theoretical results in detail. We separate the wave function into the ground state | Ψ GS › and the photo-excited component | φ ( τ )›, that is, the part of the wavefunction different from the ground state. Here | b ( τ )| 2 represents the weight of | φ ( τ )› in the total wavefunction | Ψ ( τ )›. As | φ ( τ )› includes a doublon–holon pair (see Methods), | b ( τ )| 2 is also a rough estimate of the double occupancy density. Indeed, the number of doublons left in the system at τ >0 is an order of magnitude smaller for E pump <Δ than for E pump >Δ ( Fig. 4a ), confirming that the non-adiabatic processes are less relevant for sub-gap pumping. 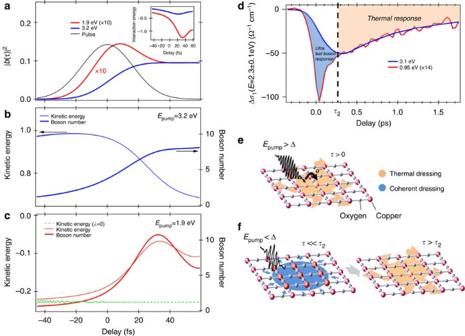Figure 4: Hubbard–Holstein calculations. (a) The weight, |b(τ)|2, of the photo-excited component of the wave function as a function of pump–probe delay for excitations below (red) and above (blue) Δ (the sub-gap weight is multiplied by 10.2, that is, it is normalized to that above gap). In the inset ofa, the interaction energy in eV is shown. The average number of bosons (thick line) and the electron kinetic energy in eV (thin line) for the two excitation wavelengths are reported inbandc. Ina,bandc, the differences between the pump-perturbed quantities and the ground state ones are shown. Ind,Fig. 2cis reproduced for clarity, with orange and blue shaded areas to underline the slow and fast responses of the bosonic field associated toEpump>Δ andEpump<Δ, respectively. Ineandf, cartoons of the physical mechanism are sketched. ForEpump>Δ (e), the dynamics is consistent with a simple thermalization or ‘thermal dressing’ scenario; forEpump<Δ (f), the ultrafast drop of kinetic energy goes in pair with the reaction of the bosonic field and a ‘coherent dressing’ mechanism is in action at very short time delays. Figure 4: Hubbard–Holstein calculations. ( a ) The weight, | b ( τ )| 2 , of the photo-excited component of the wave function as a function of pump–probe delay for excitations below (red) and above (blue) Δ (the sub-gap weight is multiplied by 10.2, that is, it is normalized to that above gap). In the inset of a , the interaction energy in eV is shown. The average number of bosons (thick line) and the electron kinetic energy in eV (thin line) for the two excitation wavelengths are reported in b and c . In a , b and c , the differences between the pump-perturbed quantities and the ground state ones are shown. In d , Fig. 2c is reproduced for clarity, with orange and blue shaded areas to underline the slow and fast responses of the bosonic field associated to E pump >Δ and E pump <Δ, respectively. In e and f , cartoons of the physical mechanism are sketched. For E pump >Δ ( e ), the dynamics is consistent with a simple thermalization or ‘thermal dressing’ scenario; for E pump <Δ ( f ), the ultrafast drop of kinetic energy goes in pair with the reaction of the bosonic field and a ‘coherent dressing’ mechanism is in action at very short time delays. Full size image To highlight the modifications driven in the system by the pump, we calculate the expectation values of different physical observables in the photo-excited state, that is, ‹ φ ( τ )| A | φ ( τ )›. The operators of interest are the kinetic energy, the number of bosons and the interaction energy. These correspond to the expectation values of H t (equation (1)), of the first part of H ebi divided by ω 0 , and of the second part of H ebi (equation (3)), respectively. These expectation values are related to the ones calculated on the total wavefunction ‹ Ψ ( τ )| A | Ψ ( τ )› through the weight | b ( τ )| 2 (see Methods for details). The interaction energy carries direct information on the interplay of the bosonic field with the excited charge carriers. Namely, this quantity is proportional to the number of bosons that are accumulated just on the site where doublons or holons are situated. For E pump >Δ, itinerant doublon–holon pairs are created ( Fig. 4a ) with a significant kinetic energy during the laser pulse ( Fig. 4b ). These pairs subsequently relax to lower energies emitting bosons on a longer timescale. The decrease of the average kinetic energy is related to the increase of the average boson number ( Fig. 4b ). The physics emerging for E pump >Δ is thus consistent with a thermalization scenario of the photo-excited doublons and holons. In the case of E pump <Δ, a completely different response is observed. During the pulse, the kinetic energy is negative both for λ =0 and for finite λ , but most important is the behaviour immediately after the pulse ( Fig. 4c ). In case of finite λ , we observe an ultrafast reaction of the bosons, which is apparent both from the maximum of the boson number at τ 1 =35 fs as well as from the minimum of the interaction energy at the same value of τ (inset of Fig. 4a ). Owing to this ultrafast reaction, the kinetic energy increases immediately after the pulse. Altogether, this is a clear signature of the ultrafast formation of strongly dressed quasi-particles. This transient state, leading to the observed optical conductivity drop around the CTP, persists for few tens of femtoseconds and only at longer times evolves into a thermal incoherent state ( τ 2 >50 fs). The time dependence of the kinetic energy and boson number ( Fig. 4c ) shows that for sub-gap pumping the energy is transferred nearly ‘instantaneously’ (on a timescale related to the inverse of the boson frequency) from the electromagnetic field into the boson subsystem through the electrons. The comparison of the kinetic energies calculated with and without the electron–boson coupling (solid and dashed lines in Fig. 4c ) indicates that the persistence of some dynamics after the end of the pump pulse for E pump <Δ is possible only with non-vanishing electron–boson interaction. In Fig. 4d we redraw for clarity the data of Fig. 2c , and cartoons of the physical mechanisms described above are shown in Fig. 4e,f for E pump >Δ and for E pump <Δ, respectively. The scenario stemming from the exact diagonalization of the Hubbard–Holstein model explains the different response measured for above-gap and sub-gap excitations. In spite of the fact that the model includes only one bosonic field, such field can be excited in a different way by the two excitation schemes. Although for E pump >Δ the boson field acts as a bath where the excess kinetic electronic energy is deposited after the excitation, sub-gap pumping triggers a quasi-instantaneous distortion of the bosonic field. It is interesting to note that for both theory and experiment the ultrafast response in the optical conductivity for E pump <Δ gives a transient feature, which is qualitatively analogous to the changes associated to a small doping ( Fig. 1c , black dashed curve). This observation leads us towards the speculation that a perturbation with sub-gap photon energy drives a non-thermal tendency to create delocalized strongly dressed quasi-particles. This discloses several possible scenarios where coherent electromagnetic fields can be used to manipulate quantum coherent phases of matter [38] , [39] . Experimental details We performed time-resolved experiments on La 2 CuO 4+ δ by combining broadband probes with ~100 fs pump pulses at different wavelengths. To address the pulse-width-limited rise time observed for E pump <Δ, we performed additional measurements with sub-20 fs pulses. The ~100 fs pump pulse measurements were performed with a Ti:Sa amplified laser at 250 kHz repetition rate. The pump energies were tuned to 0.95 eV ( E pump <Δ) and to 3.1 eV ( E pump >Δ) with durations corresponding to ~100 and ~140 fs, respectively, and about 0.04 eV bandwidth each. The 0.95 eV pulses are generated with a commercial optical parametric amplifier, the 3.1 eV pulses by second harmonic generation of the fundamental laser light in a 200-μm-thick Beta Barium Borate (BBO) crystal. The broadband probe was generated in a sapphire crystal. As expected for white-light generation [40] , the chirp of these probes is mainly linear. Thus, it has been simply corrected with the same straight line for both above-gap (~3.1 eV) and sub-gap (~0.95 eV) pump pulses. Freshly polished a – b oriented samples were mounted on the cold finger of a helium flow cryostat. The reflectivity changes Δ R ( ω , τ )= R ( ω , τ )/ R ( ω )−1 were measured in the 1.5–3.1 eV range at several temperatures between 50 and 330 K. The pump fluences of the measurements shown in Figs 2a–c and 3 are equal to 330 and 170 μJ cm −2 for the 3.1 and 0.95 eV pump pulses, respectively. These fluences correspond to about 4 × 10 −3 and 1 × 10 −3 Ph u −1 for E pump >Δ and E pump <Δ, respectively, where ph u −1 stands for photons (ph) absorbed by a chemical unit (u) of La 2 CuO 4 . The amplitude of the measured photo-induced variation of the reflectivity is linear with the pump intensity up to two times the excitation densities used in the reported experiments (see Supplementary Fig. 2 ). The sub-20 fs measurements were performed with a Ti:Sa amplified source at 1 kHz. The pump energies were tuned to 1.4 eV with 0.15 eV bandwidth ( E pump <Δ) and to 2.25 eV with 0.25 eV bandwidth ( E pump >Δ) with duration corresponding to ~12 and ~7 fs, respectively. The short pulses are obtained by compressing the output of a tunable non-collinear optical parametric amplifier with chirped mirrors or with two prisms. The measurements shown in Fig. 2d and in Supplementary Fig.1 have been performed at room temperature with pump fluences corresponding to 1.3 and 2.8 mJ cm −2 for above-gap or sub-gap pump pulses, respectively. The higher noise conditions of this set of measurements do not allow to investigate the linear response regime for the system, while the high intensities in both pump and probe pulses (≥0.2 mJ cm −2 ) are responsible for unavoidable artefacts in the transient responses. For these reasons, we limited the KK-based analysis of the optical conductivity to the long pulse measurements, which are safely in the linear response limit. Furthermore, we notice that the observed thermalization times are different for the two excitation schemes with ~100 and sub-20 fs pulses. This might be partially due to the fact that excitations produced by light pulses at certain wavelengths undergo a state-specific thermalization pathway. The longer times detected with ~100 fs pulses partially support this scenario. However, we stress that the two excitation schemes differ not only in terms of the excited states involved, but also regarding the pulse energies used, and this can affect the observed timescales. Further studies are needed to clarify this issue. Nonetheless, it is remarkable that both results confirm a pulse-width-limited non-thermal reaction of the bosonic field for E pump <Δ. Finally, we can exclude the slow rise time measured for E pump >Δ to be related to diffusion of the photo-excitation energy along the surface normal. In such case, one would expect slower rise times for shorter probe wavelengths. This effect is not observed in our experiments (see Supplementary Fig. 3 ). Thermal effects The optical response of the CTP as a function of pump–probe delay is reported in Fig. 2c for E pump >Δ (solid blue curve) and E pump <Δ (solid red curve), respectively. The transient conductivity probed at 2.3 eV for E pump =0.95 eV is properly normalized by the factor N , calculated as follows. The pump energy density absorbed by the sample and detected by a single-colour probe with energy E probe is equal to , where Ф ( E ) is the fluence, R ( E ) is the reflectivity and x ( E ) is the penetration depth for photons with energy E . Considering the bandwidth of the pump pulse and averaging over the probe energy range Δ E probe , the effective energy density is . Making use of the reflectivity and the penetration depth as determined from the ellipsometry data (see Fig. 1 and Supplementary Fig. 4b ), the ratio turns out to be ~14 at T =130 K, which is the normalization factor used in Fig. 2c . The absorbed pump energy density can be directly related to the increase of the sample temperature Δ T detected by the probe pulses. In particular, where δ denotes the mass density and C the specific heat. Being at T =130 K (ref. 41 ) and , the expected temperature reached by the sample when all the degrees of freedom thermalize is T +Δ T ≈139 K. Thus, we expect that the laser-driven transient response at long pump–probe delays should be comparable to the difference between the equilibrium optical quantities measured at 130 K and at 139 K. A comparison among the off-equilibrium Δ σ 1 ( ω , τ =5 ps) and the difference between the equilibrium conductivities σ 1 ( T =139 K) and σ 1 ( T =130 K) reveals a very good agreement, see the black dashed curves in Fig. 1c and in Fig. 3b and Supplementary Fig. 4 . The dashed line in Fig. 1c is obtained by a linear interpolation of the data in ref. 6 . Data analysis To extract the time-dependent optical quantities such as the dielectric function ( ε ) or the optical conductivity ( σ ) out of pump–probe reflectivity Δ R ( ω , τ )/ R ( ω )= R ( ω , τ )/ R ( ω )−1, we proceed as follows. We obtain the equilibrium reflectivity R ( ω ) from the measured ellipsometry data between 1 and 3.2 eV and from the literature outside of this range [6] , [42] . We perform a Drude–Lorentz fit [43] , [44] of the broadband equilibrium reflectivity over a wide energy range, from a few meV up to several tens of eV. We calculate the real and imaginary parts of the equilibrium dielectric function, ε 1 ( ω ) and ε 2 ( ω ), in the entire energy range through the KK relations [45] . The time-resolved Δ R ( ω , τ )/ R ( ω ) is measured in the 1.5–3.1 eV energy range. To obtain the time-domain changes of the optical functions, we consider only the regime where the variations of the reflectivity Δ R ( ω , τ ) (up to 10 −2 as shown in Supplementary Fig. 5 ) is linear with the pump fluence. We make the assumption that the variations of the pump-perturbed reflectivity outside the probed energy range are either small or distant on the energy scale so that they do not affect significantly the optical response in the probed range of 1.5–3.1 eV. Starting from these assumptions, both the measured reflectivity Δ R ( ω , τ )/ R ( ω ) and the equilibrium reflectivity R ( ω ) are known over a broad energy range, that is, from a few meV up to several tens of eV. Hence, the time evolution of the optical quantities such as ε 1 ( ω , τ ) and ε 2 ( ω , τ ) can be obtained by the KK transformations. The results of this analysis performed on the data measured at 130 K are reported in Fig. 2 . The photo-induced variation of the real part of the optical conductivity Δ σ 1 ( ω , τ )= σ 1 ( ω , τ )- σ 1 ( ω ) is shown for E pump =3.1 eV ( Fig. 2a ) and E pump =0.95 eV ( Fig. 2b ). We include for clarity the reflectivity data in Supplementary Fig. 5 and Supplementary Fig. 6 . We emphasize that our analysis is consistent because the same normalization factor is used in Fig. 2c (that displays Δ σ 1 ) and in Supplementary Fig. 7 (where Δ R / R is shown). We implement a transfer-matrix method to correct the effect of the mismatch between the penetration depths of the pump and the probe pulses on the amplitude of the time-domain signal. We assume a pump-perturbed exponentially graded index of refraction at the material surface by means of multiple planes, each with a thickness of 1 nm. The total reflection is calculated exploiting the continuity conditions for the electric fields across these boundaries. Further details can be found in refs 46 , 47 Being the penetration depth at ~0.95 eV larger than the one of any probe in the 1.5–3 eV range, one expects significant corrections only for E pump ~3.1 eV. The detailed numerical analysis confirms this simple picture. This is made evident in Supplementary Figs 8 and 9 for pump–probe delay time τ =0.1 ps averaged over ±0.1 ps. The Δ R ( ω , τ )/ R ( ω ) obtained in this way for E pump ~3.1 eV has been used as starting point for the KK analysis described in the previous paragraph. The corrections to the transient reflectivity are obtained as summarized in Supplementary Fig. 9 . HHH details The time-dependent potential vector adopted is [48] and the optical conductivity at time τ , after the end of the pump, is given by [49] , [50] Here , T is the time-ordering operator, j ( t ) is the current operator in the Heisenberg representation along one of the lattice axes, η is a broadening factor taking into account additional dissipative processes and M is the number of lattice sites. The | Ψ ( τ )› state is obtained through the Lanczos time-propagation method [51] . In the following, we use periodic boundary conditions on two-dimensional lattices [52] with M= 8. The local nature of the interactions involved in the HHH allows us to extract the relevant physics of the model (at least at a qualitative level) also by using a small lattice, which, on the other hand, reproduces most of the discrete symmetries of the square lattice, and contains the relevant momenta: , ( π , 0), (0, π ), (0, 0) and ( π , π ). It is worth noting that the chosen lattice does not frustrate the anti-ferromagnetic ground state [52] . These important properties are a consequence of the ‘special’ eight site lattice introduced first in ref. 53 . Within the used approach, the charge and spin degrees of freedom are exactly treated: all the possible states are considered in subspaces with a well-defined value of the z component of the total spin. The real bottleneck comes from the infinite dimensional Hilbert space required by the boson excitations. To solve this problem, we use a generalization of the method recently introduced in the Holstein [35] and Su-Schrieffer-Heeger model [34] : the double-boson approach. It is based on a smart truncation of the boson Hilbert space including two distinct sets of states. In the first set of basis elements, there are up to four bosons distributed in all possible ways. Of course, in this way the scattering processes among charge carriers and boson excitations up to four quanta are treated exactly also in q space. This set is able to recover the self-consistent Born approximation and goes beyond it, including vertex corrections. In the other set of states, local excitations of any strength (up to 15 boson excitations per site) are distributed at most on two sites, which are located at arbitrary positions with respect to the charge carriers. The double-boson approach used in this study is based on the idea that the physical properties for any value of the electron–boson interaction can be described by diagonalizing the Hamiltonian in the bosonic Hilbert subspace generated by the two sets of states introduced above (excluding obvious double counting). The pump pulses adopted in the model have slightly different temporal and energetic content with respect to the ones used in the experiments. This is mainly due to finite size effects, explained as follows. Concerning the frequency of the pump pulses, we have chosen E pump =1.9 eV and E pump =3.2 eV for sub-gap and above-gap pump pulses, respectively. In particular, for the sub-gap case, we were forced to use a larger value than that one used in the experiments for two reasons. First, solving the HHH on a small lattice implies few sparse discrete eigenstates at low energy, resulting in the lowest optical transition at ~1.9 eV that is absent in the bare Hubbard model. Second, our model does not include the free charge in excess present in the experimental sample. In addition to this, we highlight that the model is provided at T =0 K while it is well known that the CT gap in La 2 CuO 4 shifts to higher energies on cooling [30] , [31] , [32] . Moreover, the theory adopted ~40 fs long pulses, while the experiments made use of ~100 fs pulses. In the case of a small lattice, as the one used in our model, the allowed eigenvalues are restricted to a discrete set with a finite separation between them. However, due to the uncertainty principle, the more the duration of the pump pulse increases, the narrower is the energy. Hence, our model cannot use pump pulses exceeding ~40 fs, as the energy uncertainty of the pump pulses would be smaller than the typical distance between two adjacent eigenvalues. In this condition, a light pulse would excite only one eigenstate of the Hamiltonian resulting in a state not evolving in time. Nonetheless, we stress that this limit of the theory is intrinsic in the finite size of our lattice and a comparison between experiment and theory is possible as the experimental pulse will always excite a superposition of eigenstates of the system. The linearity with the pump intensity of the observed response for both experiment and theory further consolidates the validity of the comparison. In the main text, we focused our attention on the properties of | φ ( τ )›, the photo-excited component of the wave-function | Ψ ( τ )›. It is defined in terms of the wave function at time τ and | Ψ GS ›, the normalized ground state of the HHH in absence of the electromagnetic field: . The expectation value of any observable A , measured with respect to the value in the ground state wavefunction, is: , where Δ A is proportional to the matrix element of the observable between the ground state and photo-excited component. As the last term is negligible (we checked it for all the quantities investigated in the paper), the ratio between the values of any fixed physical quantity, measured in the wavefunctions corresponding to above- and sub-gap pulses, is always proportional to the ratio between the weights associated to the photo-excited components of the two wavefunctions. This ratio is about 10 for the chosen parameter values and delay larger than the pump pulse duration. Taking into account the smaller excitation fluence for the sub-gap case in the experimental data, we find a good agreement between theory and experiments. Finally, we address the role of the pump pulse duration in the Hubbard–Holstein calculations ( Supplementary Fig. 10 ). In general, one expects that for longer pump pulses the non-thermal part of the dynamical response of a system to be diminished in favour of the thermal dynamics. As the observed ultrafast shift of the transient optical conductivity is related to the non-thermal response in La 2 CuO 4+ δ for E pump <Δ, one expects that the shorter the pump pulse, the larger the shift in Δ σ 1 ( ω , τ ). This is confirmed by the calculations displayed in Supplementary Fig. 10 corresponding to ~20 fs long pump pulses, and by the experiments shown in Supplementary Fig. 1 . We stress that all the calculations predict an ultrafast transient negative change of Δ σ 1 ( ω , τ ) for E pump <Δ, that evolves towards the thermal response at long pump–probe delays. This is confirmed by both ~10 and ~100 fs resolution experiments. How to cite this article: Novelli, F. et al. Witnessing the formation and relaxation of dressed quasi-particles in a strongly correlated electron system. Nat. Commun. 5:5112 doi: 10.1038/ncomms6112 (2014).